Functional high-throughput screening identifies the miR-15 microRNA family as cellular restriction factors forSalmonellainfection Increasing evidence suggests an important role for miRNAs in the molecular interplay between bacterial pathogens and host cells. Here we perform a fluorescence microscopy-based screen using a library of miRNA mimics and demonstrate that miRNAs modulate Salmonella infection. Several members of the miR-15 miRNA family were among the 17 miRNAs that more efficiently inhibit Salmonella infection. We discovered that these miRNAs are downregulated during Salmonella infection, through the inhibition of the transcription factor E2F1. Analysis of miR-15 family targets revealed that derepression of cyclin D1 and the consequent promotion of G1/S transition are crucial for Salmonella intracellular proliferation. In addition, Salmonella induces G2/M cell cycle arrest in infected cells, further promoting its replication. Overall, these findings uncover a mechanism whereby Salmonella renders host cells more susceptible to infection by controlling cell cycle progression through the active modulation of host cell miRNAs. MicroRNAs (miRNAs) are a class of genome-encoded small RNAs that regulate eukaryotic gene expression at the post-transcriptional level, by repressing target transcripts containing partially or fully complementary binding sites present mostly in the 3′-untranslated region (UTR) and coding sequence of mRNAs [1] , [2] . Consistent with their major role in controlling gene expression, miRNAs participate in a wide range of biological processes (for example, development, cell cycle and immune response [3] , [4] , [5] ). Misregulation of miRNA expression has been linked to several pathologies, including cancer, cardiovascular diseases and immune-related disorders [4] , [6] , [7] . In addition to their well-established functions in physiological and pathological eukaryotic cell processes, it is becoming clear that miRNAs also play crucial roles during infection by viruses [8] and bacterial pathogens [9] , [10] . A role for miRNAs in the response of mammalian cells to bacterial infection was initially inferred from the observation that sensing of purified bacterial lipopolysaccharide (LPS) modulated the expression of several miRNAs, most prominently miR-155 and miR-146a/b (ref. 11 ). The first evidence of miRNA regulation as a direct consequence of bacterial infection was obtained in Arabidopsis , in which the upregulation of miR-393a triggered by the bacteria Pseudomonas syringae was shown to contribute to the resistance of the plant against the pathogen [12] . Recent efforts have focused on the identification, in mammalian cells, of miRNAs that are regulated in response to different bacterial pathogens. This analysis revealed a common set of miRNAs as the key players in the host innate immune response against bacteria, specifically miR-146, miR-155, miR-21, miR-125 and let-7. These miRNAs were shown to be regulated upon infection with various bacterial pathogens, including Helicobacter pylori , Listeria monocytogenes , Francisella tularensis , Salmonella enterica and Mycobacteria species [9] , [10] . Importantly, while the altered expression of several host miRNAs has been described as part of the immune response to bacterial infections, less is known about the functional role of miRNAs during the infection process. Salmonella enterica serovar Typhimurium (henceforth, Salmonella ) is an extensively investigated facultative intracellular bacterial pathogen, belonging to the Enterobacteriaceae family. Salmonella is one of the most common causes of gastroenteritis in humans, being a leading cause of lethality by food-borne diseases [13] . During its infection cycle, Salmonella secretes more than 30 effector proteins through two distinct type-III secretion systems (T3SS), which modulate various host cellular processes (for example, signal transduction pathways, cytoskeleton integrity, membrane trafficking and pro-inflammatory responses) [14] , [15] . Generally, secretion of effector proteins by the pathogenicity island-1 (SPI-1) T3SS occurs early during infection and is associated with the invasion of intestinal epithelial cells and biogenesis of the Salmonella -containing vacuole (SCV). The pathogenicity island-2 (SPI-2) T3SS is induced after internalization, and secretes effectors that are mainly involved in late SCV maturation, bacterial replication and intracellular survival. Salmonella infection has an impact on host miRNA expression, upregulating the well-characterized NF-kB-dependent miRNAs (miR-21, miR-146 and miR-155) in mouse macrophages, and downregulating the let-7 miRNA family both in macrophages and epithelial cells [16] . Let-7 family members repress the expression of the pro-inflammatory interleukin (IL)-6 and anti-inflammatory IL-10 cytokines and therefore let-7 downregulation upon Salmonella infection induces IL-6 and IL-10 expression, likely contributing to a balanced host inflammatory response. These results clearly highlight the relevance of the miRNA network in the regulation of Salmonella infection, and highlight the need for a more exhaustive study on the role of the miRNome on bacterial infection. The use of RNA interference screenings has improved our knowledge of the interplay between bacteria and host cells, identifying novel cellular factors critical for infection [17] , [18] , [19] . Only recently this approach has been extended to miRNAs [20] , [21] , and is yet to be applied for the identification of miRNAs critical for infection by bacterial pathogens. Here we have employed a functional, high-throughput screening approach using a genome-wide library of miRNA mimics to systematically identify miRNAs that modulate Salmonella infection of epithelial cells. We have identified 17 miRNAs that efficiently inhibit infection, several of which belonging to the miR-15 miRNA family. Interestingly, deep-sequencing analysis of miRNA expression revealed that the levels of miR-15 family members are decreased upon Salmonella infection. The identification of targets of these miRNAs that are relevant for Salmonella infection led to the characterization of the host cell cycle proteins as critical regulators of bacterial infection. In particular, we have shown that infection is not efficient in G1-arrested cells and that the downregulation of the miR-15 family by Salmonella leads to the derepression of cyclin D1, thus favouring G1/S transition and, hence, increasing intracellular bacteria proliferation. Moreover, we demonstrate that Salmonella induces G2/M arrest of the infected cells to further promote its intracellular replication, through the SpvB effector protein. Overall, our results identify a mechanism whereby Salmonella promotes its own survival and replication by modulating the levels of host cell miRNAs and the host cell cycle. Screening for miRNAs controlling Salmonella infection To identify miRNAs that are able to modulate infection by Salmonella in a systematic and comprehensive way, we performed a high-content, fluorescence microscopy-based, high-throughput screening using a library of miRNA mimics (988 mature miRNAs, 875 unique sequences, miRBase release 13.0 (2009), http://mirbase.org ; Fig. 1a ). HeLa cells, a widely used cellular model for Salmonella infection studies, were transfected with the library of miRNA mimics and after 48 h the cells were infected with a Salmonella strain containing a chromosomally integrated copy of the green fluorescent protein (GFP), at a multiplicity of infection (MOI) of 25 for 20 h. Automated image analysis was performed to quantify multiple parameters, including cell count, number of infected cells and GFP intensity ( Supplementary Fig. 1a ). The screening was performed in triplicate; the replicates showed good reproducibility (Spearman r >0.55; Supplementary Fig. 1b ). Average results from the three independent biological replicates of the screening are shown in Fig. 1b and Supplementary Fig. 1c , presented as fold change compared with control miRNA (log2 scale). On average, ~2,400 cells were analysed per well and replicate. A Caenorhabditis elegans miRNA (cel-miR-231) with no sequence homology to any known human miRNA was used as the negative control in all experiments; a short interfering RNA (siRNA) against ACTR3, a protein important for the entry of Salmonella into host cells [17] , was used as the positive control ( Supplementary Fig. 1d ). MiRNAs that decreased the cell count to less than 65% of the control were considered toxic and excluded from further analysis (180 toxic miRNAs, Supplementary Data 1 ). 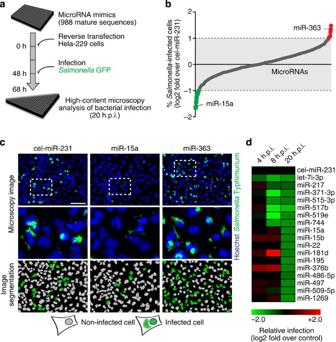Figure 1: High-content screening identifies miRNAs regulatingSalmonellainfection. (a) Schematic of screening strategy. (b) Percentage ofSalmonella-infected cells following treatment with the library of miRNA mimics.Salmonellainfection was performed at MOI 25 and analysed at 20 h.p.i. Average results from the three independent biological replicates of the screening are shown as fold change compared with the control miRNA cel-miR-231, in log2 scale. Results for 695 miRNAs are shown; 180 miRNAs decreased cell viability and were excluded. miRNAs highlighted in red and green increase or decrease infection by at least twofold, respectively. (c) Representative images of HeLa cells treated with cel-miR-231 (control), miR-15a and miR-363 (highlighted inb) and infected withSalmonella. Image analysis is shown in the bottom panel. Scale bar, 100 μm. (d) Heatmap representing the changes inSalmonellainfection, at three time points (4, 8 and 20 h.p.i., MOI 25), upon treatment with the 17 miRNAs that decreasedSalmonellainfection by at least twofold in the screening. Results are based on quantification of the percentage of infected cells and are shown as fold change compared with control miRNA. The colour scale illustrates the relative infection (log2 scale). Figure 1: High-content screening identifies miRNAs regulating Salmonella infection. ( a ) Schematic of screening strategy. ( b ) Percentage of Salmonella -infected cells following treatment with the library of miRNA mimics. Salmonella infection was performed at MOI 25 and analysed at 20 h.p.i. Average results from the three independent biological replicates of the screening are shown as fold change compared with the control miRNA cel-miR-231, in log2 scale. Results for 695 miRNAs are shown; 180 miRNAs decreased cell viability and were excluded. miRNAs highlighted in red and green increase or decrease infection by at least twofold, respectively. ( c ) Representative images of HeLa cells treated with cel-miR-231 (control), miR-15a and miR-363 (highlighted in b ) and infected with Salmonella . Image analysis is shown in the bottom panel. Scale bar, 100 μm. ( d ) Heatmap representing the changes in Salmonella infection, at three time points (4, 8 and 20 h.p.i., MOI 25), upon treatment with the 17 miRNAs that decreased Salmonella infection by at least twofold in the screening. Results are based on quantification of the percentage of infected cells and are shown as fold change compared with control miRNA. The colour scale illustrates the relative infection (log2 scale). Full size image The screening identified 17 miRNAs that strongly decreased Salmonella infection by at least twofold (green in Fig. 1b and Supplementary Fig. 1c ; Supplementary Data 1 ; 62 miRNAs by at least 1.5-fold) when compared with non-treated cells or cells treated with the control miRNA, whereas 11 miRNAs increased the infection by at least twofold (red in Fig. 1b and Supplementary Fig. 1c ; Supplementary Data 1 ). Examples of miRNAs that strongly decrease or increase Salmonella infection are shown in Fig. 1c . To better characterize the effect of the 17 miRNAs that strongly decreased infection, we determined which stage of the Salmonella infection cycle was perturbed by each miRNA, by measuring the effect of miRNA overexpression at 4 and 8 h post infection (h.p.i.). MiRNAs regulating a cellular process linked to Salmonella invasion and internalization are expected to have a prominent effect at early times post infection (4 h.p.i.). While miRNAs that affect processes linked to later steps of the infection cycle, such as maturation of the SCV or bacterial replication, are expected to affect infection only at intermediate and late times post infection (8 and 20 h.p.i., respectively). Of the 17 miRNAs tested, only let-7i-3p inhibited infection at early times post infection; overexpression of the other miRNAs decreased infection at intermediate (6 miRNAs) or late (10 miRNAs) times ( Fig. 1d ; Supplementary Fig. 1e,f ). Overall, these results identify a subset of miRNAs that inhibit Salmonella infection by interfering with cellular pathways critical for different stages of the bacteria infection cycle. miR-15 family inhibits Salmonella infection Among the 17 miRNAs decreasing Salmonella infection by at least twofold were four of the eight members of the miR-15 miRNA family (miR-15a, miR-15b, miR-195, miR-497). Importantly, all members of this miRNA family (miR-15a, miR-15b, miR-16, miR-195, miR-424, miR-497, miR-503 and miR-646; Fig. 2a ) decreased infection by at least 1.5-fold ( Fig. 2b,c ; Supplementary Data 1 ). However, miR-646 decreased the viability of HeLa cells and was therefore excluded. The inhibitory effect of the miR-15 family on Salmonella infection was validated using several alternative approaches: (i) quantification of the GFP levels in infected cells using quantitative reverse transcriptase–PCR (qRT–PCR; Supplementary Fig. 2a ); (ii) colony-forming unit (CFU) assay ( Supplementary Fig. 2b ); and (iii) analysis of the percentage of GFP-positive cells using flow cytometry ( Supplementary Fig. 2c ). Of note, miR-15 family members did not increase host cell membrane permeability, which could have potentially enabled gentamicin access to the intracellular bacteria, compared with control miRNA ( Supplementary Fig. 2d ). 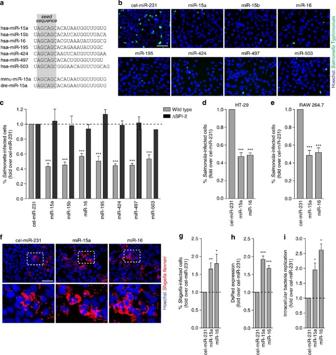Figure 2:Salmonellainfection is inhibited by the miR-15 family. (a) Sequences of the mature forms of the human miR-15 family members. Mouse (mmu) and zebrafish (dre) miR-15a are shown for comparison. Seed sequence is highlighted. (b) Representative images of HeLa cells treated with members of the miR-15 family or control miRNA (cel-miR-231) and infected withSalmonella. Scale bar, 100 μm. (c) Percentage of HeLa cells infected withSalmonellawild-type or ΔSPI-2 strains, after treatment with members of the miR-15 family. (d) Percentage of HT-29 and (e) RAW 264.7 cells infected withSalmonellaupon treatment with control miRNA, miR-15a or miR-16. (f) Representative images of HeLa cells treated with control miRNA, miR-15a or miR-16 and infected withShigella. Scale bar, 100 μm. (g) Percentage of HeLa cells infected withShigella, (h) DsRed expression quantified using qRT–PCR and (i) CFU quantification upon treatment with control miRNA, miR-15a or miR-16.SalmonellaandShigellainfections were performed at MOI 25 (HeLa and HT-29) or MOI 10 (RAW 264.7) and analysed at 20 h.p.i. Results are normalized to control miRNA and shown as mean±s.e.m. *P<0.05, **P<0.01, ***P<0.001, two-tailed Student’st-test;n≥3. Figure 2: Salmonella infection is inhibited by the miR-15 family. ( a ) Sequences of the mature forms of the human miR-15 family members. Mouse (mmu) and zebrafish (dre) miR-15a are shown for comparison. Seed sequence is highlighted. ( b ) Representative images of HeLa cells treated with members of the miR-15 family or control miRNA (cel-miR-231) and infected with Salmonella . Scale bar, 100 μm. ( c ) Percentage of HeLa cells infected with Salmonella wild-type or ΔSPI-2 strains, after treatment with members of the miR-15 family. ( d ) Percentage of HT-29 and ( e ) RAW 264.7 cells infected with Salmonella upon treatment with control miRNA, miR-15a or miR-16. ( f ) Representative images of HeLa cells treated with control miRNA, miR-15a or miR-16 and infected with Shigella . Scale bar, 100 μm. ( g ) Percentage of HeLa cells infected with Shigella , ( h ) DsRed expression quantified using qRT–PCR and ( i ) CFU quantification upon treatment with control miRNA, miR-15a or miR-16. Salmonella and Shigella infections were performed at MOI 25 (HeLa and HT-29) or MOI 10 (RAW 264.7) and analysed at 20 h.p.i. Results are normalized to control miRNA and shown as mean±s.e.m. * P <0.05, ** P <0.01, *** P <0.001, two-tailed Student’s t -test; n ≥3. Full size image Time course infection experiments revealed that members of the miR-15 family decrease infection only at 20 h.p.i. ( Figs 1d and 2b,c ; Supplementary Figs 1e,f and 2e,f ), suggesting that these miRNAs are affecting host cell pathways necessary for Salmonella replication, but not related to entry or early steps of infection. In agreement with these results, the miR-15 family did not inhibit infection by the Salmonella ΔSPI-2 mutant strain, which invades target cells but is defective in intracellular replication ( Fig. 2c ; Supplementary Fig. 2g,h ). Considering that Salmonella infects a variety of host target cells, both phagocytic and non-phagocytic, we assessed the inhibitory effect of the miR-15 family in two other cell lines commonly used for Salmonella infection studies: HT-29 cells, a human intestinal epithelial infection model, and murine RAW 264.7 cells, which has macrophage-like characteristics. The tested miR-15 family members inhibited Salmonella infection in both HT-29 ( Fig. 2d ; Supplementary Fig. 2i–k ) and RAW 264.7 cells ( Fig. 2e ; Supplementary Fig. 2l–n ), demonstrating that the effect of miR-15 on Salmonella infection is not cell type-specific, but rather a general and conserved phenomenon. To establish whether inhibition of infection by the miR-15 family is common to other bacterial pathogens, we analysed the effect of this miRNA family on the infection by Shigella flexneri , an enteroinvasive pathogen closely related to Salmonella . Surprisingly, overexpression of miR-15 family members significantly increased infection by Shigella , as shown with high-content microscopy, qRT–PCR and CFU assay ( Fig. 2f–i ). These results indicate that the miR-15 family restricts Salmonella infection by regulating a host cell pathway(s) critical for the intracellular replication of Salmonella , but is dispensable for Shigella . Salmonella infection downregulates miR-15 family To compare the findings from the high-throughput screening analysis with the changes in miRNA expression occurring during infection, we performed deep-sequencing analysis of cDNA libraries prepared from the small RNA population (10–29 nt) isolated from HeLa cells infected with Salmonella (20 h.p.i.) and mock-treated cells. Considering that at an MOI of 25 Salmonella is internalized in only 10–15% of the HeLa cells, we separated the fraction of cells that had internalized Salmonella ( Salmonella +) from the bystander fraction ( Salmonella −) by fluorescence-activated cell sorting (FACS), and analysed miRNA levels within these samples. We observed that Salmonella infection decreased overall miRNA expression. Interestingly, all miR-15 family members were significantly downregulated upon Salmonella infection ( Fig. 3a ). This was particularly evident in the Salmonella + fraction of infected cells. 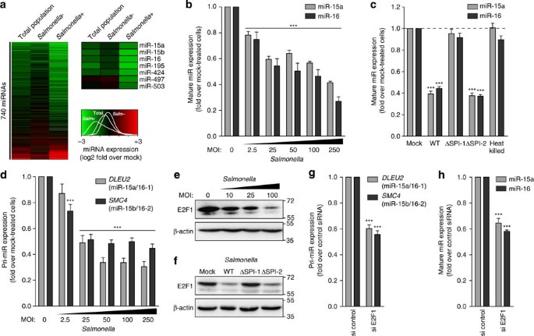Figure 3: miR-15 family expression is downregulated bySalmonellainfection. (a) Changes in miRNA expression uponSalmonellainfection (MOI 25) of HeLa cells. Results are shown for total population, fraction of cells with internalizedSalmonella(Salmonella+) and bystander fraction (Salmonella−). Only miRNAs with number of reads ≥25 in the mock-treated sample are shown. The inset shows expression of the miR-15 family members. The colour scale illustrates the frequency of miRNA expression (log2 scale) for the different cell populations (total,Salm− andSalm+). (b,c) Expression of mature miR-15a and miR-16 determined by qRT–PCR in HeLa cells infected with (b)Salmonellawild type at the indicated MOIs or (c) mutant strains defective in invasion (ΔSPI-1, MOI 100), intracellular replication (ΔSPI-2, MOI 100) or heat-killedSalmonella(MOI 100). (d) Quantification of miR-15 pri-miRNA transcripts using qRT–PCR in HeLa cells infected withSalmonellaat the indicated MOIs. miR-15a/miR-16-1 and miR-15b/miR-16-2 are processed fromDLEU2andSMC4transcripts, respectively. (e,f) E2F1 expression determined using western blot upon infection with (e)Salmonellawild type at the indicated MOIs or (f) mutant strains defective in invasion (ΔSPI-1, MOI 100) or intracellular replication (ΔSPI-2, MOI 100). (g,h) Expression of (g) pri-miRNAs and (h) mature forms of miR-15 family members upon knockdown of E2F1, determined using qRT–PCR in HeLa cells. Samples were collected at 20 h.p.i. Results are shown as mean±s.e.m., normalized to mock-treated cells (b–d) or control siRNA (g,h). ***P<0.001, two-tailed Student’st-test;n≥3. Figure 3: miR-15 family expression is downregulated by Salmonella infection. ( a ) Changes in miRNA expression upon Salmonella infection (MOI 25) of HeLa cells. Results are shown for total population, fraction of cells with internalized Salmonella ( Salmonella +) and bystander fraction ( Salmonella− ). Only miRNAs with number of reads ≥25 in the mock-treated sample are shown. The inset shows expression of the miR-15 family members. The colour scale illustrates the frequency of miRNA expression (log2 scale) for the different cell populations (total, Salm − and Salm +). ( b,c ) Expression of mature miR-15a and miR-16 determined by qRT–PCR in HeLa cells infected with ( b ) Salmonella wild type at the indicated MOIs or ( c ) mutant strains defective in invasion (ΔSPI-1, MOI 100), intracellular replication (ΔSPI-2, MOI 100) or heat-killed Salmonella (MOI 100). ( d ) Quantification of miR-15 pri-miRNA transcripts using qRT–PCR in HeLa cells infected with Salmonella at the indicated MOIs. miR-15a/miR-16-1 and miR-15b/miR-16-2 are processed from DLEU2 and SMC4 transcripts, respectively. ( e,f ) E2F1 expression determined using western blot upon infection with ( e ) Salmonella wild type at the indicated MOIs or ( f ) mutant strains defective in invasion (ΔSPI-1, MOI 100) or intracellular replication (ΔSPI-2, MOI 100). ( g,h ) Expression of ( g ) pri-miRNAs and ( h ) mature forms of miR-15 family members upon knockdown of E2F1, determined using qRT–PCR in HeLa cells. Samples were collected at 20 h.p.i. Results are shown as mean±s.e.m., normalized to mock-treated cells ( b – d ) or control siRNA ( g , h ). *** P <0.001, two-tailed Student’s t -test; n ≥3. Full size image Downregulation of miR-15 family members upon Salmonella infection was confirmed using qRT–PCR specific for mature miRNAs, and shown to be MOI-dependent ( Fig. 3b ; Supplementary Fig. 3a ), likely reflecting an increase in Salmonella + cells. Downregulation was also time-dependent: at early and intermediate times of infection the mature miR-15 miRNAs were slightly decreased compared with mock-treated cells (4 and 8 h.p.i. ; Supplementary Fig. 3b ), whereas a clear downregulation was observed at 20 h.p.i. ( Fig. 3b ; Supplementary Fig. 3a ). To identify the stimulus responsible for the downregulation of the miR-15 family upon Salmonella infection, we first treated HeLa cells with purified Salmonella LPS, tumour necrosis factor alpha (TNFα) and heat-killed Salmonella . These different stimuli did not induce changes in miR-15 levels ( Fig. 3c ; Supplementary Fig. 3c,d ), in agreement with the lack of expression in HeLa cells of Toll-like receptor (TLR) 2, TLR5 and the TLR4 co-factor MD-2 (refs 22 , 23 ), which have been implicated in the recognition of various pathogen-associated molecular patterns including LPS and flagellin. Next we assessed the effect of infection with Salmonella mutant strains defective in invasion (ΔSPI-1) or intracellular replication (ΔSPI-2) on expression of miR-15 family. Interestingly, infection with the Salmonella ΔSPI-2 strain caused a strong downregulation of the miR-15 family, comparable to wild type (WT), whereas the ΔSPI-1 strain did not affect miR-15 family expression ( Fig. 3c ; Supplementary Fig. 3c ). Collectively, these data demonstrate that, during infection, Salmonella overcomes restriction by the miR-15 family members by downregulating their expression and that this effect is dependent on host cell invasion. Salmonella infection inhibits transcription of miR-15 family To understand whether Salmonella -induced regulation of the miR-15 family occurs at the level of miRNA biogenesis or stability, we investigated the changes of the relevant pri-miRNAs using qRT–PCR. We observed that the pri-miRNAs corresponding to miR-15a/miR-16-1 and miR-15b/miR-16-2 ( DLEU2 and SMC4 genes, respectively) progressively decreased with increasing Salmonella MOIs ( Fig. 3d ). Infection with the Salmonella ΔSPI-2 strain caused downregulation of the pri-miRNA expression, comparable to WT, whereas the invasion-defective ΔSPI-1 strain showed no effect ( Supplementary Fig. 3e ). The downregulation of the miR-15 pri-miRNAs correlated with the decreased levels of the corresponding mature miRNAs (compare Fig. 3b,d ), although the decrease in pri-miRNA levels at early and intermediate times of infection (4 and 8 h.p.i. ; Supplementary Fig. 3f ) preceded the reduction in mature miRNAs. These results suggest that transcription inhibition of the miR-15 family members upon Salmonella infection is the cause of decreased mature miRNA expression. Previously, it has been reported that members of the miR-15 family are under the direct transcriptional control of E2F1 (ref. 24 ), a transcription factor best known for its regulation of the gene expression programme required for cell cycle progression. E2F1 binds to the promoters of DLEU2 and SMC4 genes leading to increased expression of the miRNAs that are processed from these genes. We analysed E2F1 expression upon Salmonella infection and observed that E2F1 mRNA and protein levels decrease in an MOI-dependent manner ( Fig. 3e ; Supplementary Fig. 3g ). In agreement with the regulation of miR-15 expression, the decrease in E2F1 was dependent on Salmonella internalization ( Fig. 3f ; Supplementary Fig. 3h ). Importantly, knockdown of E2F1 downregulates miR-15 family expression, both at the pri-miRNA and mature miRNA levels ( Fig. 3g,h ; Supplementary Fig. 3i ). Overall, these data demonstrate that Salmonella infection decreases E2F1 expression and as a consequence downregulates the miR-15 family. Cyclin D1 is required for Salmonella infection To obtain a global picture of the targets of the miR-15 family, we assessed transcriptome changes in HeLa cells transfected with three members of the miR-15 family (miR-15a, miR-16 or miR-503) or a control miRNA (cel-miR-231) using deep sequencing. We observed an extensive overlap of the genes downregulated by these three miRNAs, as expected for miRNAs belonging to the same family ( Supplementary Fig. 4a ). In total, 876 genes were downregulated by these miRNAs (reads ≥25 for control miRNA, average 1.5-fold downregulation; Fig. 4a ; Supplementary Data 2 ), which likely include their direct targets. 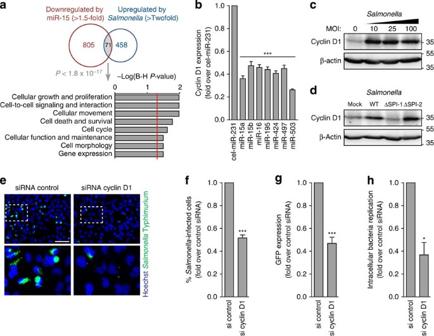Figure 4: Cyclin D1 is required forSalmonellainfection. (a) Overlap between genes downregulated upon overexpression of miR-15 family members (miR-15a, miR-16 and miR-503; average ≥1.5-fold) and genes upregulated bySalmonellainfection (twofold or more; MOI 100). Functional categories enriched among the 71 overlapping genes are shown. Enrichment analysis was performed using IPA, applying Benjamini–Hochberg multiple testing correction; the eight most enriched categories are shown. Red line representsP=0.05. (b) Cyclin D1 expression determined using qRT–PCR upon overexpression of members of the miR-15 family. (c,d) Cyclin D1 expression determined using western blot upon infection with (c)Salmonellawild type at the indicated MOIs or (d) mutant strains defective in invasion (ΔSPI-1, MOI 100) or intracellular replication (ΔSPI-2, MOI 100). (e) Representative images of HeLa cells treated with control siRNA or cyclin D1 siRNA, and infected withSalmonella(MOI 25). Scale bar, 100 μm. (f) Percentage of HeLa cells infected withSalmonella, (g) GFP expression determined using qRT–PCR and (h) CFU quantification upon treatment with control siRNA or cyclin D1 siRNA.Salmonellainfection was analysed at 20 h.p.i. Results are shown as mean±s.e.m., normalized to control miRNA (cel-miR-231;b) or control siRNA (f–h). *P<0.05, ***P<0.001, two-tailed Student’st-test;n≥3. Figure 4: Cyclin D1 is required for Salmonella infection. ( a ) Overlap between genes downregulated upon overexpression of miR-15 family members (miR-15a, miR-16 and miR-503; average ≥1.5-fold) and genes upregulated by Salmonella infection (twofold or more; MOI 100). Functional categories enriched among the 71 overlapping genes are shown. Enrichment analysis was performed using IPA, applying Benjamini–Hochberg multiple testing correction; the eight most enriched categories are shown. Red line represents P =0.05. ( b ) Cyclin D1 expression determined using qRT–PCR upon overexpression of members of the miR-15 family. ( c , d ) Cyclin D1 expression determined using western blot upon infection with ( c ) Salmonella wild type at the indicated MOIs or ( d ) mutant strains defective in invasion (ΔSPI-1, MOI 100) or intracellular replication (ΔSPI-2, MOI 100). ( e ) Representative images of HeLa cells treated with control siRNA or cyclin D1 siRNA, and infected with Salmonella (MOI 25). Scale bar, 100 μm. ( f ) Percentage of HeLa cells infected with Salmonella , ( g ) GFP expression determined using qRT–PCR and ( h ) CFU quantification upon treatment with control siRNA or cyclin D1 siRNA. Salmonella infection was analysed at 20 h.p.i. Results are shown as mean±s.e.m., normalized to control miRNA (cel-miR-231; b ) or control siRNA ( f – h ). * P <0.05, *** P <0.001, two-tailed Student’s t -test; n ≥3. Full size image In addition, we evaluated the transcriptome changes induced by infection with Salmonella (20 h.p.i., MOI 100). This analysis revealed 680 genes downregulated and 529 genes upregulated (reads ≥25 for mock-treated cells, twofold regulation; Fig. 4a ; Supplementary Data 2 ). Since Salmonella infection induces the downregulation of the miR-15 family, it is reasonable to assume that miR-15 targets will be derepressed upon Salmonella infection. Therefore, to identify putative miR-15 family target genes relevant for controlling Salmonella infection, we compared the genes downregulated by miR-15 family with those upregulated upon Salmonella infection. We identified 71 genes that fulfilled both these criteria ( Fig. 4a ; Supplementary Data 2 ). Functional analysis of these genes revealed enrichment for genes belonging to the ‘cellular growth and proliferation’ and ‘cell cycle’ categories ( Fig. 4a ). Among the genes in these two enriched functional categories, we focused our attention on cyclin D1 ( CCND1 ), a protein with a central role in the regulation of cell cycle and cell proliferation [25] , and a validated target of several miR-15 family members [26] , [27] . We extended this analysis and validated that all members of miR-15 family downregulate cyclin D1 ( Fig. 4b ). Most importantly, we measured cyclin D1 levels during infection and confirmed that cyclin D1 is strongly upregulated, both at the protein and mRNA levels ( Fig. 4c and Supplementary Fig. 4b ). This regulation was dependent on bacterial internalization ( Fig. 4d and Supplementary Fig. 4c ) and cyclin D1 inversely correlated with miR-15 expression, being significantly increased at intermediate and late times of infection (8 and 20 h.p.i. ; Fig. 4c and Supplementary Fig. 4b,d ) when the downregulation of miR-15 by Salmonella is more pronounced. Importantly, knockdown of cyclin D1 is sufficient to inhibit Salmonella infection ( Fig. 4e–h , Supplementary Fig. 4e ), recapitulating the effect observed with miR-15 family mimics. Cyclin D1 knockdown did not change host cell membrane permeability compared with control siRNA ( Supplementary Fig. 4f ). A similar decrease in Salmonella infection was observed in HT-29 cells upon cyclin D1 knockdown ( Supplementary Fig. 4g–j ). These results demonstrate that, by downregulating the miR-15 family, Salmonella infection increases cyclin D1 expression, which is required for efficient infection. Salmonella infection is inhibited in G1 phase-arrested cells Cyclin D1 is a main determinant of the G1/S phase transition [25] . During the G1 phase, cyclin D1 interacts with CDK4 or CDK6 kinases initiating the phosphorylation of the retinoblastoma family of transcriptional repressors. This allows the release of the E2F transcription factors, which promote the transcription of genes required for entry into the S phase. To determine whether the effect of cyclin D1 on Salmonella infection is a direct consequence of its role in the cell cycle, we measured the efficiency of Salmonella infection in G1-arrested HeLa cells. HeLa cells were blocked in G1 by using an inhibitor of CDK4/6 kinases (CDK4/6 inhibitor IV, CDK4/6i; Supplementary Fig. 5a,b ). Although no differences in Salmonella infection were observed in G1-arrested cells compared with control cells at early times post infection (4 h.p.i. ; Supplementary Fig. 5c,d ), a strong decrease in infection was observed at later times (20 h.p.i. ; Fig. 5a–c ; Supplementary Fig. 5e ), in agreement with the results obtained for cyclin D1 knockdown and the miR-15 family mimics. These results were further corroborated by a significant decrease in Salmonella infection observed in cells depleted of CDK4 or CDK6 ( Fig. 5a–c ). Treatment with CDK4/6i did not affect host cell membrane permeability ( Salmonella+ fraction; Supplementary Fig. 5f ). 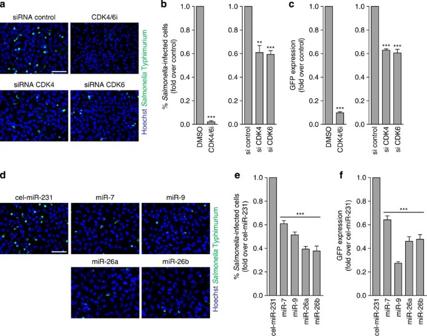Figure 5: The G1 phase of the host cell cycle is detrimental forSalmonellaintracellular replication. (a) Representative images of HeLa cells treated with an inhibitor of CDK4/6 (CDK4/6i, 10 μM) or with siRNAs against CDK4 or CDK6, and infected withSalmonella. Scale bar, 100 μm. (b) Percentage of HeLa cells infected withSalmonellaand (c) GFP expression quantified using qRT–PCR upon CDK4/6 inhibitor, or CDK4 or CDK6 siRNA treatment. (d) Representative images of HeLa cells treated with control miRNA, miR-7, miR-9, miR-26a or miR-26b and infected withSalmonella. Scale bar, 100 μm. (e) Percentage of HeLa cells infected withSalmonellaand (f) GFP expression quantified using qRT–PCR upon transfection of the selected miRNAs shown ind.Salmonellainfection was performed at MOI 25 and analysed at 20 h.p.i. Results are shown as mean±s.e.m., normalized to DMSO or control siRNA (b,c) or control miRNA (e,f). **P<0.01, ***P<0.001, two-tailed Student’st-test;n≥3. Figure 5: The G1 phase of the host cell cycle is detrimental for Salmonella intracellular replication. ( a ) Representative images of HeLa cells treated with an inhibitor of CDK4/6 (CDK4/6i, 10 μM) or with siRNAs against CDK4 or CDK6, and infected with Salmonella . Scale bar, 100 μm. ( b ) Percentage of HeLa cells infected with Salmonella and ( c ) GFP expression quantified using qRT–PCR upon CDK4/6 inhibitor, or CDK4 or CDK6 siRNA treatment. ( d ) Representative images of HeLa cells treated with control miRNA, miR-7, miR-9, miR-26a or miR-26b and infected with Salmonella . Scale bar, 100 μm. ( e ) Percentage of HeLa cells infected with Salmonella and ( f ) GFP expression quantified using qRT–PCR upon transfection of the selected miRNAs shown in d . Salmonella infection was performed at MOI 25 and analysed at 20 h.p.i. Results are shown as mean±s.e.m., normalized to DMSO or control siRNA ( b , c ) or control miRNA ( e , f ). ** P <0.01, *** P <0.001, two-tailed Student’s t -test; n ≥3. Full size image Knowing that miRNAs can inhibit Salmonella infection by arresting host cells in G1, we investigated whether other miRNAs identified in the screening could act through a similar mechanism. Interestingly, among the miRNAs that significantly inhibited Salmonella infection by at least 1.5-fold in the screening we found several miRNAs that have been reported to inhibit G1/S transition, namely miR-7, miR-9, miR-26a and miR-26b [28] , [29] , [30] . We validated the effect of these miRNAs on Salmonella infection ( Fig. 5d–f ). Of note, cell cycle analysis confirmed that treatment with mimics of these miRNAs, as well as with members of the miR-15 family or cyclin D1 siRNA, triggered G1 delay in HeLa cells ( Supplementary Fig. 5g–j ), whereas overexpression of cyclin D1 results in a faster progression to S and G2 phases of the cell cycle ( Supplementary Fig. 5k,l ). Altogether, these results demonstrate that the G1 phase of the host cell cycle is detrimental for the intracellular proliferation of Salmonella . G2/M arrest of host cells favors Salmonella infection Bacterial pathogens can manipulate the host cell cycle in different ways to their own advantage. While certain pathogens block cell cycle progression indiscriminately, others arrest cell cycle specifically in G1 (for example, Neisseria gonorrhoeae [31] , Helicobacter pylori [32] ) or G2/M phases (for example, S. flexneri [33] , Staphylococcus aureus [34] ). Given our results showing that Salmonella infection is impaired in G1-arrested cells and that infection leads to upregulation of cyclin D1 via miR-15 downregulation, thereby promoting G1/S transition, we hypothesized that Salmonella replication might be favoured in the G2/M phase. Indeed, G2 arrest of HeLa or HT-29 cells by treatment with RO-3306, an inhibitor of CDK1 (ref. 35 ), resulted in a strong increase in intracellular replication of Salmonella ( Fig. 6a–c , Supplementary Figs 5a,b and 6a–c ). 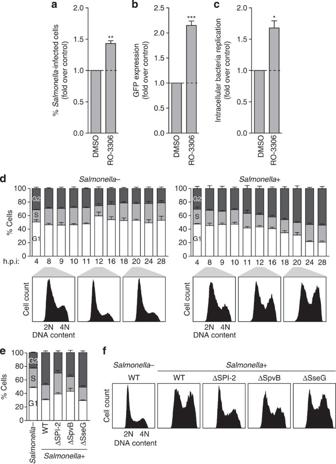Figure 6:Salmonellainfection arrests host cells in the G2/M phase of the cell cycle. (a) Percentage of HeLa cells infected withSalmonella(MOI 25), (b) GFP expression determined using qRT–PCR and (c) CFU quantification upon treatment with DMSO (control) or RO-3306 (9 μM), an inhibitor of CDK1. Samples were collected at 14 h.p.i. (d) Percentage of HeLa cells in the different stages of the cell cycle uponSalmonellainfection (MOI 50) at the indicated times post infection. Analysis is shown for fraction of cells with internalizedSalmonella(Salmonella+) and the bystander fraction (Salmonella−). Cell cycle stage distribution was determined using FACS, following propidium iodide staining. Representative cell cycle profiles for 8, 12 and 20 h.p.i. are shown. Population of cells in G2 is significantly increased inSalmonella+ compared withSalmonella− fractions, from 12 h.p.i. onwards (P<0.05, two-tailed Student’st-test). (e) Percentage of HeLa cells in the different stages of the cell cycle, and (f) representative cell cycle profiles, upon infection with wild-type (MOI 100) and different mutantSalmonellastrains (MOI 250). Analysis is shown for fraction of cells with internalizedSalmonella. Bystander population from the cells treated with wild-typeSalmonella(Salmonella−) is shown for comparison. Population of cells in G2 for theSalmonella+ fraction is significantly decreased in ΔSPI-2 and ΔSpvB, compared with WT (P<0.05, two-tailed Student’st-test). Data are shown as mean±s.e.m. 2Nand 4Nind,eindicate cells having diploid or tretraploid DNA content, respectively. *P<0.05, **P<0.01, ***P<0.001, two-tailed Student’st-test;n≥3. Figure 6: Salmonella infection arrests host cells in the G2/M phase of the cell cycle. ( a ) Percentage of HeLa cells infected with Salmonella (MOI 25), ( b ) GFP expression determined using qRT–PCR and ( c ) CFU quantification upon treatment with DMSO (control) or RO-3306 (9 μM), an inhibitor of CDK1. Samples were collected at 14 h.p.i. ( d ) Percentage of HeLa cells in the different stages of the cell cycle upon Salmonella infection (MOI 50) at the indicated times post infection. Analysis is shown for fraction of cells with internalized Salmonella ( Salmonella +) and the bystander fraction ( Salmonella −). Cell cycle stage distribution was determined using FACS, following propidium iodide staining. Representative cell cycle profiles for 8, 12 and 20 h.p.i. are shown. Population of cells in G2 is significantly increased in Salmonella + compared with Salmonella − fractions, from 12 h.p.i. onwards ( P <0.05, two-tailed Student’s t -test). ( e ) Percentage of HeLa cells in the different stages of the cell cycle, and ( f ) representative cell cycle profiles, upon infection with wild-type (MOI 100) and different mutant Salmonella strains (MOI 250). Analysis is shown for fraction of cells with internalized Salmonella . Bystander population from the cells treated with wild-type Salmonella ( Salmonella −) is shown for comparison. Population of cells in G2 for the Salmonella + fraction is significantly decreased in ΔSPI-2 and ΔSpvB, compared with WT ( P <0.05, two-tailed Student’s t -test). Data are shown as mean±s.e.m. 2 N and 4 N in d , e indicate cells having diploid or tretraploid DNA content, respectively. * P <0.05, ** P <0.01, *** P <0.001, two-tailed Student’s t -test; n ≥3. Full size image To investigate whether, in the normal context of infection of epithelial cells, Salmonella has an impact on host cell cycle progression, HeLa cells were infected with Salmonella and the cell cycle distribution was analysed over time for cells with internalized Salmonella ( Salmonella +) and the bystander fraction ( Salmonella −). Although an increase in cells in the G2/M phase could be detected as early as 12 h.p.i. for the Salmonella + compared with Salmonella − or mock-treated cells, this effect was more striking at late times post infection (20 to 28 h.p.i., Fig. 6d , Supplementary Fig. 6d,e ). To better characterize this effect, cells were synchronized in late G1 by double thymidine block and then infected with Salmonella and simultaneously released from the block. A delay of Salmonella + cells in G2 was observed in the first round of the cell cycle (compare 10–12 h post release for mock-treated or Salmonella − and Salmonella + cells; Supplementary Fig. 6f,g ), with a more pronounced block observed at later stages (20–28 h.p.i. ; Supplementary Fig. 6f,g ). Detailed analysis of the kinetics of G2/M arrest induced by Salmonella infection revealed that this effect is more prominent at late times post infection, indicating that it might be associated with SPI-2 T3SS activity. In favour of this hypothesis, the Salmonella ΔSPI-2 strain resulted in significantly less G2/M arrest of the infected cells than WT Salmonella ( Fig. 6e,f , Supplementary Fig. 7a,b ). More than 20 Salmonella proteins are translocated by the SPI-2 T3SS into the host cell cytoplasm, subverting multiple host pathways/functions. To determine which of these proteins might induce G2/M arrest, we screened a collection of effector gene mutants for their effect on host cell cycle. Most of the mutant strains induced G2/M arrest to the same extent as the WT Salmonella ( Supplementary Table 1 ). However, infection with the ΔSpvB mutant resulted in a host cell cycle profile similar to the ΔSPI-2 strain ( Fig. 6e,f ; Supplementary Fig. 7a,b ). In agreement with our observation that G2/M arrest promotes infection, the ΔSpvB strain replicated slightly, but significantly, less efficiently than the WT strain [36] (~70% of WT, Supplementary Fig. 7c ). Of note, mutants that infect with an efficiency lower than ΔSpvB still induced G2/M arrest (for example, ΔSseG; Fig. 6e,f ; Supplementary Fig. 7a–c ), arguing against the possibility that the lower replication rate of the ΔSpvB mutant impairs its ability to cause G2/M arrest. Identical results were obtained in HT-29 cells ( Supplementary Fig. 7d,e ). Overall, these results show that Salmonella causes arrest of the infected cells in the G2/M phase of the cell cycle, through the activity of the SpvB effector, to promote its intracellular proliferation. Bacterial pathogens have developed sophisticated mechanisms to subvert the key host cell pathways to establish a productive infection. Considering the pervasive role of miRNAs in the control of gene expression and their involvement in numerous biological processes, the premise that miRNAs are the major players in the interaction between the host and bacterial pathogens is of particular interest. Indeed, miRNAs have been extensively described as part of the immune response to various bacterial pathogens, from plants to vertebrates (reviewed in refs 9 , 10 , 37 ). However, considerably less is known regarding miRNAs that functionally regulate bacterial infections and whether bacterial pathogens are also able to exploit host miRNAs to promote their own intracellular survival and proliferation. The present study is the first to address these questions on a genome-wide level, using a combination of high-throughput functional screening with a library of miRNA mimics and miRNA profiling by deep sequencing. Salmonella Typhimurium was used as a model bacterial pathogen for these studies. Our results show that host miRNAs can strongly modulate infection by Salmonella , and that different miRNAs interfere with distinct steps of the infection cycle. Of the 875 tested miRNAs, we identified 17 miRNAs that decrease and 11 miRNAs that increase Salmonella infection by at least twofold. Among the miRNAs restricting infection by Salmonella , we identified the miR-15 miRNA family. Interestingly, we also observed that Salmonella infection downregulates the miR-15 family at the transcriptional level, through the downmodulation of the transcriptional activator E2F1. Importantly, the expression of E2F3 is not affected by Salmonella infection ( Supplementary Fig. 3j ). E2F3 has been shown to be sufficient for cell proliferation and normal embryonic and post-natal development [38] , [39] , [40] , thus explaining the observed cell cycle progression despite the downregulation of E2F1 by Salmonella . Of note, downregulation of the miR-15 family is not triggered by sensing of extracellular bacteria, since LPS as well as the Salmonella ΔSPI-1 invasion mutant failed to induce miR-15 regulation, but it is rather dependent on Salmonella invasion of target cells. The exact trigger of this downregulation is yet to be identified. These results show an active role of Salmonella in downregulating host miRNAs that counteract infection, and reveal host miRNAs, in particular the miR-15 miRNA family, as a new class of host antibacterial factors that are targeted by Salmonella to achieve a productive infection. By comparing genes that are downregulated upon overexpression of miR-15 family members and genes upregulated upon Salmonella infection, we identified cyclin D1 as one of the miR-15 target that plays a key role in Salmonella infection. The involvement of the mir-15 family in controlling G1/S transition by regulating multiple cell cycle-related genes has been previously established [41] . In fact, cyclin D1, an essential factor for G1/S cell cycle progression, was shown to be a direct target of several members of the miR-15 family [26] , [27] . The observations that knockdown of cyclin D1, CDK4 or CDK6 and treatment with a CDK4/6 inhibitor fully recapitulate the phenotype observed with the miR-15 family establish a causal relationship between G1 arrest and the inhibitory effect of miR-15 family on Salmonella infection. This is further supported by our results showing that other miRNAs that induce G1 arrest (for example, miR-7, miR-9, miR-26a and miR-26b) also block infection by Salmonella . Therefore, the downregulation of the miR-15 family and consequent derepression of cyclin D1 (and potentially other cell cycle-related targets) triggered by Salmonella internalization promotes the G1/S transition of the infected cells and entry into a cell cycle stage that is more favourable for bacterial intracellular replication. It is becoming increasingly clear that some bacteria have evolved specialized strategies to interfere with the cell cycle of host cells, particularly through the use of bacterial toxins and effectors, generally termed cyclomodulins [42] . For example, cytolethal distending toxins (CDTs) are a class of heterotrimeric toxins produced by diverse unrelated Gram-negative pathogenic bacteria, including Escherichia coli , Shigella dysenteriae , Campylobacter spp., Salmonella typhi , Haemophilus ducreyi and Helicobacter hepaticus [43] . These toxins were initially shown to trigger G2/M arrest in mammalian cells, but further studies with the E. coli CDT have shown that it can also induce cell cycle arrest in G1. The CDT-mediated cell cycle arrest was shown to be linked to DNA damage cascade activation. The cycle-inhibiting factors of enteropathogenic and enterohaemorrhagic E. coli have also been shown to induce host cell cycle arrest in G1 and G2, through the stabilization of the cyclin-dependent kinase inhibitors p21 and p27 (ref. 44 ). Shigella flexneri was shown to induce G2/M arrest of epithelial cells, by a mechanism mediated by the effector protein IpaB through the targeting of Mad2L2 (ref. 33 ), an inhibitor of the anaphase-promoting complex. In addition to proteins, miRNAs have also been shown to be involved in the regulation of cell cycle during bacterial infection. H. pylori has been shown to induce cell cycle arrest of gastric cells at the G1/S transition [32] , which is in part explained by the decrease in miR-372 and miR-373 expression upon infection, leading to the post-transcriptional release of LATS2 (ref. 45 ), a regulator of cell cycle progression. It remains unclear whether the G1/S arrest of gastric cells induced by H. pylori is beneficial or detrimental for infection. Our data identify the Salmonella SpvB effector protein as being responsible for inducing G2/M arrest of infected cells. The SpvB protein, an effector encoded by the Salmonella virulence plasmid, is delivered into the host cytosol via the SPI-2 T3SS and has been shown to induce actin depolymerization via its ADP-ribosyltransferase activity [46] , [47] , [48] . Considering that compounds that interfere with actin polymerization have been shown to induce G2/M arrest [49] , [50] , it is conceivable that the effect of SpvB on cell cycle progression is connected to its actin depolymerization activity. Of note, these results are in agreement with a recent report showing that ectopic overexpression of SpvB induces cell cycle arrest in different cell lines [51] . Notwithstanding the various reports of bacterial pathogens that interfere with the host cell cycle, presumably for the pathogen’s benefit, the consequences to their infection cycle remain, in most cases, unclear. While some studies suggest that slowing down or arresting the cell cycle might be used by bacteria to perturb the integrity of the epithelial barrier and therefore allow access to the subepithelial layer, others indicate that this may constitute a countermeasure of bacterial pathogens to prevent rapid epithelial turnover [52] , [53] . According to the latter, epithelial cells would be maintained as a replicative reservoir, particularly relevant in the case of infections of the gastric and intestinal epithelia. Our data, showing that Salmonella infection is specifically inhibited in the G1 phase and that intracellular bacterial proliferation is favoured in G2/M-arrested cells, argue in favour of a critical role of the host cell cycle during Salmonella infection. This is supported by Salmonella using two distinct mechanisms to drive the host cell cycle ( Fig. 7 ): (i) the active downregulation of the miR-15 family and the consequent enforcement of the G1/S transition via derepression of cell cycle-related miR-15 targets, most prominently cyclin D1, and (ii) the G2/M arrest induced by the SpvB effector protein. In agreement with a preference of Salmonella for G2/M cells, Santos et al . [54] recently showed that Salmonella preferentially invades mitotic cells and linked this effect to an increase in cholesterol levels in the plasma membrane of the host cells. Further work is necessary to determine the reason for the cell cycle stage preference for Salmonella replication. 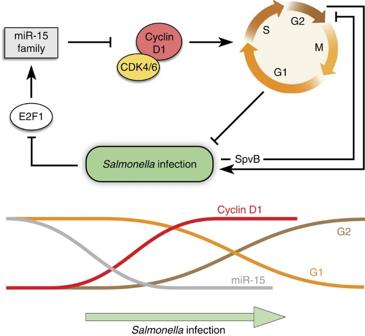Figure 7: Role of the miR-15 family in the interplay betweenSalmonellaand the host cell. IntracellularSalmonellaproliferation is inhibited in host cells in the G1 phase of the cell cycle. During infection,Salmonellainduces the downregulation of the miR-15 family, through E2F1, and the consequent derepression of its cell cycle-related targets, most prominently cyclin D1, thus promoting the passage through the G1/S transition. In addition,SalmonellaSpvB effector protein induces G2/M arrest of infected cells, thus maintaining the cells in a cell cycle stage more favourable for bacterial replication. Figure 7: Role of the miR-15 family in the interplay between Salmonella and the host cell. Intracellular Salmonella proliferation is inhibited in host cells in the G1 phase of the cell cycle. During infection, Salmonella induces the downregulation of the miR-15 family, through E2F1, and the consequent derepression of its cell cycle-related targets, most prominently cyclin D1, thus promoting the passage through the G1/S transition. In addition, Salmonella SpvB effector protein induces G2/M arrest of infected cells, thus maintaining the cells in a cell cycle stage more favourable for bacterial replication. Full size image This study constitutes the first demonstration that Salmonella can manipulate host cell functions through the modulation of host miRNA expression, with the ultimate goal of rendering the cell more susceptible to infection. Cell culture Human epithelial HeLa-229 (ATCC) cells were grown in DMEM 1 g l −1 glucose (Life Technologies) supplemented with 10% fetal bovine serum (Biochrom). Human HT-29 (ATCC) and mouse RAW 264.7 (ATCC) cells were grown in RPMI 1640 (Life Technologies) supplemented with 10% fetal bovine serum. All cell lines were maintained in a 5% CO 2 , humidified atmosphere, at 37 °C. Bacterial strains Salmonella enterica serovar Typhimurium strain SL1344 constitutively expressing GFP from a chromosomal locus and Shigella flexneri serotype 5 strain M90T expressing DsRed from a plasmid are referred to as WT throughout this work. Salmonella WT and mutant strains have been described previously [36] . Salmonella and Shigella were grown aerobically in Luria Broth (LB) or Trypticase Soy broth, respectively. Where appropriate, liquid and solid media were supplemented with antibiotics (100 μg ml −1 ampicillin or 20 μg ml −1 chloramphenicol). miRNA and siRNA transfection The library of miRNA mimics (miRIDIAN miRNA mimics) corresponding to all the human mature miRNAs (988 miRNAs, 875 unique sequences, miRBase 13.0) was obtained from Dharmacon, Thermo Scientific. MiRNA mimics are synthetic molecules that are designed so that one of the strands of the duplex is identical to the mature miRNA sequence of the miRNA of interest and therefore is able to mimic its biological activities; the complementary strand is chemically modified to avoid incorporation into the RISC complex and can thus be considered biologically inert. For the miRNA screening, miRNAs were transferred robotically from stock library plates to 384-well plates (Viewplate-384 black, clear bottom, PerkinElmer). MiRNAs were transfected into HeLa-229 cells using a standard reverse transfection protocol, at a final miRNA concentration of 50 nM. Briefly, the transfection reagent (Lipofectamine RNAiMAX, Life Technologies) was diluted in OPTI-MEM (Life Technologies) and added to the miRNAs arrayed on 384-well plates; 30 min after, 1.5 × 10 3 cells were seeded per well. Forty-eight hours after transfection, cells were infected with Salmonella (MOI 25), as described below. Cells were fixed at 20 h.p.i. and counterstained with HCS CellMask Deep Red stain (1:15,000; Life Technologies) and Hoechst 33342 (1:5,000; Life Technologies), according to the manufacturer’s instructions. Transfection was optimized using a toxic siRNA targeting ubiquitin C (UBC), which results in the death of virtually all cells ( Supplementary Fig. 1c ). The screening was performed in triplicate at the ICGEB High-Throughput Screening Facility ( http://www.icgeb.org/high-throughput-screening.html ). For RNA isolation and CFU assays, transfection experiments were performed in 24-well plates. The selected miRNAs or siRNAs were transfected as described above, except that 5.0 × 10 4 cells were seeded per well. CDK4, CDK6, CCND1 and E2F1 predesigned siRNAs were purchased from Sigma (Cat no. SASI_Hs01_00122490, SASI_Hs01_00048792, SASI_Hs01_00213909 and SASI_Hs01_00162220, respectively). UBC and ACTR3 human siGENOME SMARTpools were purchased from Dharmacon, Thermo Scientific (Cat no. M-012077-01 and M-019408-01, respectively); siGENOME Non-Targeting siRNA 5 (Dharmacon, Thermo Scientific) was used as the negative control. HT-29 and RAW 264.7 cells were transfected as described above for HeLa-229 cells, at a final miRNA concentration of 50 and 100 nM, respectively. HT-29 cells and RAW 264.7 cells were seeded in 24-well plates, at a density of 8.0 × 10 4 cells and 1.0 × 10 5 per well, respectively. Bacterial infections Overnight cultures of Salmonella or Shigella were diluted 1:100 in fresh L-broth medium and grown aerobically until OD 2 or 0.4, respectively. Bacteria were harvested by centrifugation and resuspended in complete medium. HeLa-229 cells were infected with Salmonella at MOI 25 for the screening and all microscopy-based experiments. Shigella infection was performed at MOI 25. For the RNA isolation, protein extracts and CFU assays, cells were infected at the indicated MOIs. After addition of bacteria, cells were centrifuged at 250 g for 10 min at room temperature (RT) followed by 20 min incubation at 37 °C in 5% CO 2 , humidified atmosphere. The medium was then replaced with fresh medium containing gentamicin (50 μg ml −1 ) to kill extracellular bacteria. Following 30-min incubation, the medium was replaced with fresh medium containing 10 μg ml −1 gentamicin for the remaining of the experiment. Unless otherwise indicated, cells were collected 20 h after infection. To quantify Salmonella and Shigella intracellular replication (CFU assay), infected cells were thoroughly washed with phosphate-buffered saline (PBS) and lysed with PBS containing 0.1% Triton-X-100. Samples were then serially diluted in PBS and plated on LB plates. The number of colonies formed from the recovered bacteria was counted and compared with that obtained from the input bacteria used for infection. Image acquisition and analysis Image acquisition was performed using an ImageXpress Micro automated high-content screening fluorescence microscope (Molecular Devices) at a × 20 magnification; a total of 16 images were acquired per wavelength, well and replicate, corresponding to ca . 2,400 cells analysed per well and replicate. Image analysis was performed using the ‘Multi-Wavelength Cell Scoring’ application module implemented in MetaXpress software (Molecular Devices). Briefly, nuclei and cells were segmented based on the Hoechst and CellMask stainings, respectively, and cells were then classified as positive or negative for Salmonella , depending on the total area of Salmonella staining (GFP). In addition to the percentage of infected cells, the GFP intensities after treatment with each of the tested miRNAs, which we used as a surrogate for the amount of intracellular bacteria, were measured. Given the very strong linear correlation between the percentage of infected cells and the amount of intracellular bacteria (GFP intensity; Spearman r =0.87), the analysis of Salmonella infection was performed based on the first, more informative, parameter. We have defined a threshold of cell viability at 65% and miRNAs that decreased the cell number of host cells to less than 65% of the control were considered toxic and excluded from further analysis; 180 miRNAs were excluded based on this criterion. LPS, TNFα and heat-killed Salmonella stimulation For LPS and TNFα stimulation, HeLa cells were seeded in 24-well plates (5.0 × 10 4 cells per well) and treated 48 h later with LPS (Sigma, L6143) at 1 μg ml −1 and 10 μg ml −1 or with TNFα (Sigma, T6674) at 10 ng ml −1 and 20 ng ml −1 for 20 h and then collected for RNA isolation. For heat-killed Salmonella stimulation, bacteria were prepared as described above, except that before infection, bacteria were washed twice in PBS, incubated for 2 h at 80 °C and then resuspended in complete medium. Infection was performed under the same conditions as for live bacteria and the cells were collected 20 h later for RNA isolation. Infection with live bacteria was performed in parallel as control. RNA isolation and quantitative real-time PCR Total RNA, including small RNA fraction, was extracted using miRNeasy Mini Kit (Qiagen), according to the manufacturer’s instructions. For quantification of gene expression, total RNA was reverse-transcribed using hexameric random primers followed by qRT–PCR using SsoAdvanced SYBR Green Supermix (Bio-Rad), according to the manufacturer’s instructions. The following primer pairs were used: GFP 5′- ATGCTTTTCCCGTTATCCGG -3′ and 5′- GCGTCTTGTAGTTCCCGTCATC -3′; DsRed 5′- TCATCTACAAGGTGAAGTTC -3′ and 5′- AGCCCATAGTCTTCTTCT -3′; E2F1 5′- GCAGAGCAGATGGTTATG -3′ and 5′- TGAAAGTTCTCCGAAGAGT -3′; CCND1 5′- AGGAGAACAAACAGATCA -3′ and 5′- CGGATTGGAAATGAACT T-3′; DLEU2 5′- AAGTAGCAGCACATAATG -3′ and 5′- TTAGAATCTTAACGCCAATA -3′; SMC4 5′- GATTCTCTTATTCTTGTTACTT -3′ and 5′- TAATGATTCGCATCTTGA -3′; 18S 5′- GACAGGATTGACAGATTG -3′ and 5′- ATCGGAATTAACCAGACA -3′ and beta-actin 5′- CCTGTACGCCAACACAGTGC -3′ and 5′- ATACTCCTGCTTGCTGATCC -3′. Expression was normalized to 18S or beta-actin. For miRNA quantification, RNA was transcribed using miRCURY LNA Universal cDNA synthesis kit (Exiqon) followed by qRT–PCR using predesigned miRCURY LNA PCR primer sets (Exiqon) and miRCURY LNA SYBR Green master mix (Exiqon), according to the manufacturer’s instructions. Expression of selected miRNAs was normalized to SNORD44 or hsa-miR-29a-3p. Fold changes were determined using the 2−ΔΔ C t method. RNA sequencing Library preparation and deep sequencing were performed by Vertis Biotechnology AG. Briefly, total RNA samples were fragmented using ultrasound (four pulses of 30 s each). RNAs <20 nt were removed using the Agencourt RNAClean XP kit (Beckman Coulter Genomics). The RNA samples were then poly(A)-tailed using poly(A) polymerase, and the 5′triphosphate and eukaryotic cap structures were removed using tobacco acid pyrophosphatase. Afterwards, an RNA adapter was ligated to the 5′-monophosphate of the RNA. First-strand cDNA synthesis was performed using an oligo(dT)-adapter primer and M-MLV reverse transcriptase. The resulting cDNAs were PCR-amplified to ~20–50 ng μl −1 using a high-fidelity DNA polymerase. The primers used for PCR amplification were designed for TruSeq sequencing according to Illumina instructions. The cDNAs were purified using the Agencourt AMPure XP kit (Beckman Coulter Genomics) and were analysed with capillary electrophoresis. For the preparation of the libraries for miRNA analysis, the small RNA fractions (10–29 nt) were isolated from the total RNA samples using Caliper LabChip XT apparatus. The remaining steps of the library preparation were performed as described above. For the transcriptomic analysis, six samples were pooled in equimolar amounts, and the cDNA pool was eluted in the size range of 150–600 bp from a preparative agarose gel. For the miRNA analysis, 12 samples were pooled and eluted in the size range of 155–180 bp from a polyacrylamide gel. One pool was loaded on one lane of an Illumina flowcell and clusters created by Illumina cBot. The clusters were sequenced on an Illumina HiSeq2000 using 100 cycles. Computational RNA-Seq analysis After demultiplexing of the sequences, adapter sequences were removed from the reads in fastq format. The reads were quality-trimmed using the fastq_quality_trimmer tool (from the FastX suite version 0.0.13) with a cutoff Phred score of 20 and converted to fasta format using fastq_to_fasta (FastX suite). Further read processing, including polyA-tail removal, size filtering (minimal length 12 nt after clipping), statistics generation, coverage calculation and normalization, was performed with the RNA-analysis pipeline READemption [55] version 0.1.5 using default parameters. Segemehl version 0.1.3 (ref. 56 ) was used for the read alignment and DESeq 1.12.1 (ref. 57 ) for differential gene expression analysis. For the transcriptomic analysis of cells infected with Salmonella and for miR-15 family overexpression, reads were mapped against the whole human genome (build hs37d5, 1,000 Genome project). For miRNA expression analysis, reads were aligned to the mature miRNA sequences provided by miRBase (release 20), and only reads that mapped to the miRNA reference sequences were used for differential gene expression analysis. The demultiplexed files and coverage files in wiggle format have been deposited in NCBI’s Gene Expression Omnibus and are accessible through GEO Series accession number GSE53281 . Functional gene analysis Functional analysis of the genes commonly downregulated by miR-15 family members and the genes upregulated upon Salmonella infection was conducted using the Ingenuity Pathway Analysis Software (IPA, Ingenuity Systems). Data sets were uploaded into IPA and analysed for functional enrichment in terms of ‘Molecular and Cellular Functions’, based on the information in the Ingenuity Knowledge Base. Enrichments were calculated by IPA using multiple hypothesis correction based on the Benjamini–Hochberg method; corrected P values are shown. Whole-cell protein extracts and western blot Cells were washed with PBS and harvested into 1 × Laemmli’s sample buffer. Protein samples were separated in 10% SDS–PAGE, followed by western blotting. The following antibodies were used: E2F1 (Santa Cruz, SC-251, 1:500), cyclin D1 (Invitrogen, 33–3500, 1:200), β-actin (Sigma, A2228, 1:5,000). Anti-mouse secondary antibodies coupled to horseradish peroxidase (1:5,000, GE Healthcare) were used. Signals were detected using SuperSignal West Dura Extended Duration Substrate (Pierce, 34075) and an ImageQuant LAS 4000 CCD camera (GE Healthcare). The uncropped images of immunoblots can be found in Supplementary Fig. 8 . Cell synchronization Double thymidine synchronization: HeLa cells were seeded in six-well plates (3 × 10 5 cells) and, after 9 h, were treated with 2 mM thymidine (Sigma, T1895). Cells were released from the first thymidine block after 14 h by three washes with fresh medium. Nine hours later, cells were blocked a second time with 2 mM thymidine for 16 h. Cells were released by three washes with fresh medium and directly infected with Salmonella WT at MOI 50. Cells were then collected at 4, 8, 9, 10, 11, 12, 16, 18, 20, 24 and 28 h post release; non-synchronized cells were used as control for each time point. Cells were washed once in PBS, fixed for 15 min at RT in 4% paraformaldehyde, washed twice in PBS and permeabilized in 70% ethanol at −20 °C for at least 16 h. G1 arrest: cells seeded in six-well plates (3 × 10 5 HeLa cells, 4 × 10 5 HT-29 cells) or in 24-well plates (5 × 10 4 HeLa cells, 7 × 10 4 HT-29 cells) were treated after 36 h with an inhibitor of the CDK4 and CDK6 kinases, CDK4/6 Inhibitor IV (CDK4/6i; Merck Millipore, 219492), at 10 μM or with dimethylsulphoxide (DMSO) as control. The cells were infected 16 h later with Salmonella (at MOI 50 or 100 for HeLa or HT-29 cells, respectively) in presence of the inhibitor. After 20 h, cells for cell cycle analysis were collected and fixed as described for the double thymidine synchronization; cells for microscopy analysis, CFU assays and RNA isolation were collected as described above. G2 arrest: HeLa and HT-29 cells were seeded as described above. HeLa cells were treated 48 h after seeding with 9 μM of a CDK1 kinase inhibitor, RO-3306 (Sigma, SML0569) or with DMSO as control, infected 9 h later in presence of the inhibitor with Salmonella WT at MOI 50 and collected 14 h post infection, as described above. HT-29 cells were treated 36 h after seeding with 4.5 μM of RO-3306 or with DMSO as control, infected 16 h later in presence of the inhibitor with Salmonella WT at MOI 100 and collected 20 h post infection, as described above. Nocodazole synchronization: HeLa cells (1.5 × 10 5 cells) were reverse-transfected with miRNA mimics (50 nM) or siRNA (25 nM) in 12-well plates as described above. For overexpression of HA-tagged cyclin D1, HeLa cells (5 × 10 5 cells) were seeded into 6-cm dishes 24 h before transfection. The cells were transfected using FuGENE HD Transfection reagent (Promega, E2311) with either 2 μg of pRc/CMV-CyclinD1-HA [58] (Addgene, plasmid 8948) or 2 μg of pAS1B-HA [59] plasmid in combination with 0.2 μg of pBabe/GEM2 (ref. 60 ) plasmid, which expresses an internal membrane-anchored GFP, as a transfection marker. After 24 h, the cells were trypsinized and transferred into six-well plates (miRNA and siRNAs) or 10-cm dishes (plasmids). The cells were treated the following day with 0.1 μg ml −1 nocodazole (Sigma, M1404) for 18 h (siRNA), 14 h (miRNA) or 8 h (plasmids). Cells were then harvested, washed once in PBS and fixed in 70% ethanol at −20 °C for at least 16 h. Flow cytometry and cell sorting For cell cycle analysis, cells were fixed as described above and washed with PBS and DNA staining was performed for 30 min at 37 °C with 50 μg ml −1 propidium iodide (Sigma, P4170) and 0.2 mg ml −1 RNAse A (Sigma, R5503) in buffer H (20 mM HEPES, 160 mM NaCl, 1 mM EGTA). Cells were analysed on a FACSCalibur apparatus (Becton Dickinson) and data analysis of the distribution of the different phases of cell cycle was performed using the FlowJo software (Tree Star Inc) with the Dean-Jett-Fox model. At least 15,000 live singlet cells were considered for each subpopulation. For assessment of infection rates, cells harvested in PBS 0.05 M EDTA were pooled with their supernatant in order to collect potentially detached cells, centrifuged for 5 min at 550 g at 4 °C, washed twice in ice-cold PBS and resuspended in ice-cold buffer (10 mM HEPES/NaOH, 140 mM NaCl and 2.5 mM CaCl 2 ). Cells were then analysed on a FACSCalibur apparatus (Becton Dickinson) and at least 10,000 GFP-positive cells were acquired for each condition. For measurement of cell permeability, cells were collected as described above and incubated for 15 min at RT in buffer (10 mM HEPES/NaOH, 140 mM NaCl and 2.5 mM CaCl 2 ) with 5 μl 7-Amino-Actinomycin (BD Biosciences, 51-68981E), a viable dye unable to cross intact cell membranes. Cells were kept on ice until analysis on a FACSCalibur apparatus and at least 10,000 cells were considered for each subpopulation ( Salmonella− and Salmonella+ ). For cell sorting, HeLa cells were seeded in six-well plates (3 × 10 5 cells) and infected 48 h later with Salmonella WT (MOI 25) as described above. At 20 h after infection, cells were trypsinized and collected in PBS. Sorting of the GFP-negative cells ( Salmonella− ) and GFP-positive cells ( Salmonella+ ) was performed using a FACSAria III flow cytometer (BD Biosciences) based on the signal intensity from the FITC-A channel. Mock-treated cells were also subjected to the same procedure. Sorted cells (6 × 10 5 cells for each fraction) were collected in 2 ml tubes and further processed for RNA isolation as described above. Statistical analysis All data are presented as mean±s.e.m. Statistical analysis was carried out using the Prism Software (GraphPad). For statistical comparison of two groups, two-tailed paired Student’s t -test was used. A value of P <0.05 was considered significant. Statistical significance of the overlap between two groups of genes was calculated using hypergeometric probability. How to cite this article: Maudet, C. et al . Functional high-throughput screening identifies the miR-15 microRNA family as cellular restriction factors for Salmonella infection. Nat. Commun. 5:4718 doi: 10.1038/ncomms5718 (2014). Accession codes: Data are deposited at GEO, under accession number GSE53281 .